Delay-induced anomalous fluctuations in intracellular regulation Direct negative feedback decreases fluctuations and is a ubiquitous mechanism for homoeostatic control. However, intracellular regulation frequently operates indirectly, resulting in delayed responses. Here we derive an analytical expression that quantifies the consequences from delayed negative feedback resulting from typical multistep synthesis pathways, for example, transcription or translation. We find that indirect feedback leads to more fluctuations than without feedback for intermediate delays, but surprisingly not for long delays. The anomalous fluctuations at intermediate delays emerge from positive correlations between the delayed regulatory events, and are shown to be equivalent to an increased stoichiometry in the synthesis of new molecules. The results primarily give us insight about the design principles of delayed stochastic control systems and why a fixed feedback delay gives more fluctuations than a broadly distributed feedback delay. It is also shown that the feedback delay of auto-repressed regulators can result in more sensitive regulation of downstream processes through stochastic focusing. All macro molecules and most metabolites in the cell are synthesized through a series of intermediate biochemical steps. Their production is commonly feedback regulated to sustain homoeostasis and to suppress the always present intrinsic fluctuations resulting from the birth and death of individual molecules. The biochemical feedback mechanisms do, however, also obey the probabilistic laws of biochemistry as they are realized through chemical reactions between noisy components, which may hamper the fidelity of the feedback response [1] . In addition, the feedback regulation is usually indirect, acting early in the process leading to the final product, which is desirable as formation of intermediate products are avoided when being in excess. The downside is that such indirect feedback will result in a delayed response equivalent to the time needed to synthesize the intermediate molecules. As the chemical steps are stochastic, the synthesis time will be different for each molecule even under stationary conditions, whereas the distribution of the feedback delay time will be well defined. However, the delay distribution can be different for different growth conditions, as the rates of intermediary events will depend on, for example, the availability of nutrients and enzymes. A well-known example is that amino-acid starvation alters the synthesis rates of proteins [2] , [3] , [4] . Naturally occurring regulatory networks have evolved to deal with regulatory delays, as well as changes in the distributions of delay times, and to understand the rationale in their operation. Quantitative modelling and analysis have to take the same considerations. On the modelling side, there are different approaches to investigate indirect feedback regulation. It is desirable to reduce the dimensionality of the problem, keeping it tractable without losing important dynamical properties. Therefore, unless only a very few synthesis steps are modelled, the steps are frequently collapsed and replaced by an explicit—fixed—delay in the feedback, which is formally correct in the limit of many steps [5] , [6] . In addition, it is often attractive to reduce the dimensionality by formulating the models in the limit of many molecules, in which the average concentration of molecules can be modelled with differential equations [7] . In these limits, it is well known that the delayed feedback may result in large amplitude oscillations [8] , [9] , where the feedback system is out of phase with species it is trying to regulate. Such delay-induced oscillations are, for example, believed to drive specific molecular clocks [10] , [11] . For feedback regulation in systems with a limited number of molecules, the intrinsic noise in the chemical reactions has to be analysed in combination with the delayed feedback. In these cases, stochastic kinetics with delayed reactions can be straightforwardly simulated [12] , [13] with small modifications of the stochastic simulation algorithm [14] . Such Monte Carlo approaches can be used to investigate dynamic properties for specific models and parameters, but give limited insights into the general principles for how stochastic kinetics of homoeostatic control or other biochemical feedback networks are influenced by delays. In this paper, we quantify the noise properties of general delayed feedback by starting from the individual reactions leading to the delayed response. As will be shown, the delayed feedback will not only result in decreased relaxation rates but also in a positively correlated synthesis activity. Fluctuations arising from correlated synthesis events will have a maximum for feedback delays longer than the lifetime of the regulated quantity and result in a noise level higher than unregulated synthesis. In addition, we will show that this phenomenon is not correctly retained in a model where a fixed feedback delay is replacing the indirect regulation of the multistep synthesis. 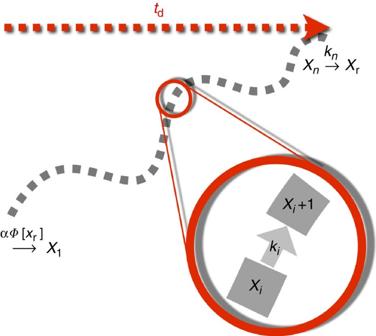Figure 1: Illustration of a multistep synthesis with indirect feedback regulation. Xiis the number of molecules of stateiandkithe transition rate from stateitoi+1.Φis the feedback, which controls the flow of molecules into the first state.Xris the number of final molecules regulated by the indirect feedback. The average time for making thensteps istd. Multistep and delay dynamics We can picture a general multistep synthesis chain similar to the illustration in Figure 1 . Each step i corresponds to one chemical state or molecular species, which is transferred chemically or physically to the next state in the chain with the rate k i . The n steps could, for instance, be the individual transcription events in polymerizing a regulatory RNA molecule. The number of molecules in the final state X r —the 'r-molecule'—is the quantity that is monitored and regulated through a feedback mechanism controlling the influx of molecules into the first state X 1 . The r-molecule is finally degraded with the rate b . The feedback Φ = Φ [ x r ] is an arbitrary function of the concentration of the regulated molecule x r and captures the processing of the regulatory control. It can take any shape, with the only restriction being 0≤ Φ ≤1—maximal influx a whenever Φ =1 and no influx when Φ =0. For an autorepressor, Φ could be the Hill function, describing that the fraction of time regulatory sites are bound by X r , but can be more intricate depending on the complexity of the feedback control. The model contains n +1 variables, and we use the shorthand notation, step feedback model, 'SFM', when referring to this model. Frequently, the individual steps are replaced with a finite delay t d in the feedback response, equivalent to the mean synthesis time. Then, the model only contains one variable, the number of r-molecules. The argument of the feedback function is in this setting translated to the concentration of the r-molecule at time t − t d . We abbreviate this model as the delay feedback model, 'DFM'. Figure 1: Illustration of a multistep synthesis with indirect feedback regulation. X i is the number of molecules of state i and k i the transition rate from state i to i +1. Φ is the feedback, which controls the flow of molecules into the first state. X r is the number of final molecules regulated by the indirect feedback. The average time for making the n steps is t d . Full size image Let us first express the equations describing the SFM and DFM in the limit of a large number of well-stirred molecules. For practical reasons, we rescale time with the lifetime of the r-molecule, 1/ b , which gives us time τ = bt , maximal influx α = a / b and step rate κ i = k i / b . The (dimensionless) equations then read with . The solution x r satisfying the delay differential equation, describing the dynamics of the DFM is a good approximation of x r in (1), when the number of steps n is large ( Supplementary Note 1 ). Both (1) and (2) have the same stationary solution x r,s given by αΦ [ x r,s ]= x r,s , which is stable to perturbations for certain combinations of feedback delays and (logarithmic) feedback gains , which is a measure of the relative change in synthesis rate per relative change in X r at the steady state x r,s . The system becomes oscillatory when the feedback gain is too strong in relation to the feedback delay, that is, if the regulation responds too strongly based on old information, it is easy to overshoot to goal (ref. 15 and Supplementary Note 1 ). Molecular fluctuations The fluctuations originating in the biochemical reactions can be analysed by the chemical master equation [16] , describing the changes in probability for occupying each chemical state. Unfortunately, we can only calculate the noise properties exactly from the chemical master equation in very simple cases [17] , [18] , and usually we have to rely on approximation methods. An often used route is the linear noise approximation (LNA) [16] that can be used to estimate mean values and the covariances of copy number fluctuations. The covariance C ij between two species i and j in the LNA satisfies Lyapunov's matrix equation at the stable stationary solution x s where A is the Jacobian matrix describing the linearized dynamics around steady state and V the diffusion matrix. Both A and V are specified in the Methods section. We are interested in the variance of the X r -molecule, C rr . For a constant κ i = κ , i= 1,..., n , we have τ d = n / κ and C rr can be calculated by a recursive relation of the elements in (3) ( Supplementary Note 2 ): The term is non-negative and defined as the stoichiometric delay coefficient for reasons that will be explained in the next section. As the feedback gain φ appears both in the numerator and the denominator of C rr , it may potentially increase or decrease the variance, depending on the feedback delay τ d = t d / b . γ is a variable with a maximal magnitude of the order of unity that can be determined in various limits. Production of (single) molecules without feedback gives a variance that follows the mean, corresponding to a Poisson process. Any other value of the variance is an effect of the feedback gain and the feedback delay. The stoichiometric delay coefficient We will now explain the origin of the stoichiometric delay coefficient by starting with a simple example. Suppose that we have two reactions where molecules are created and annihilated and the average in- and out-flux of molecules are constant, but that we have some freedom in designing the stoichiometry. A simple example would be to have a reaction where one molecule is created, on average, every second, with the alternative to create two molecules every other second. The two alternatives are equal in the macroscopic description, but differ if molecular fluctuations are considered [16] . Formally, suppose that each birth step generates p molecules and that molecules decay individually. The rates of production and decay are given by f [ x ] and g [ x ], respectively, In the LNA (3), the variance of X is given by the rate of reaction events multiplied by their stoichiometries squared divided by the rate of relaxation to steady state, that is, where f s = f [ x s ] and g s = g [ x s ] at the steady state x s , and we in the last row assume constant production and spontaneous decay. The average number of molecules 〈 X 〉= x s . Molecular fluctuations thus increase linearly with the stoichiometry p . If each reaction creates one molecule, p =1, we obtain Poissonian statistics. Let us now apply the same ideas to the creation and annihilation of r-molecules in the SFM and the DFM. Assume for a moment that the feedback delay occasionally leads to synthesis of several new molecules during a short interval, because multiple delayed synthesis events are initiated before the number of molecules changes and synthesis is downregulated. The impact of creating two molecules in two successive events, much closer in time than the average time between synthesis events, is equivalent to one reaction where two molecules are created. Such close synthesis events can therefore be interpreted as an average increase in stoichiometry, p =1+ s d . The coefficient s d = s d [ τ d ] is a—yet to be determined—function of the feedback delay that we call the stoichiometric delay coefficient. Assuming that the effects of the delayed feedback can be described by a change in the stoichiometry and relaxation rate for a one species system, X r , we end up with the following birth and death scheme: with , as equally many molecules are, on average, created regardless of the change in the stoichiometry—at equilibrium we have the in- and out-flux . Repeating the calculations from the p -stoichiometry example earlier (7), with the relaxation (the denominator) given by the eigenvalues of the Jacobian of the SFM and the DFM (calculated in Supplementary Note 1 ), yields the expressions we obtained in (4a) and (4b), respectively. We thus conclude that the term s d is a result of a delay altered stoichiometry, hence the name stoichiometric delay coefficient. The stoichiometric delay coefficient can be estimated for different feedback gains and feedback delays from equation (5). When the feedback delay is small, defined by , the stoichiometric delay coefficient scales linearly with the feedback delay ( Supplementary Note 2 ) Note also that the increase is independent of the number of biochemical steps n . The linear increase in this regime is because of an increased accumulation of positively correlated synthesis events. For large feedback delays, (implying a finite n ) and small feedback gains, , the stoichiometric delay coefficient can be approximated as ( Supplementary Note 2 ) In this limit, the coefficient is decreasing with the feedback delay and now depends on the number of biochemical steps n . The decrease with increasing is in this case because of the broadening of the distribution of the feedback delay, which will be clarified shortly. Combining equation (9) and equation (10), we conclude that for feedback gains that cannot induce oscillations the stochiometric delay coefficient attains its maximum for finite feedback delays. 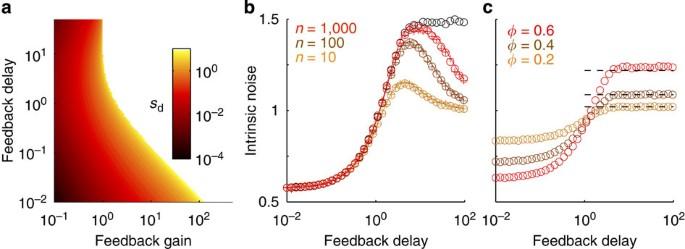Figure 2: Feedback-regulated molecular fluctuations. (a) The size of the stoichiometric delay coefficientsdfor different feedback gains and feedback delays in the SFM withn=100. Macroscopic oscillations of the concentration appear with parameters in the white area. (b,c) Intrinsic noise measured by the Fano factor of the SFM and the DFM. In (b), the solid line is the LNA, the plus signs stochastic simulations of the SFM and the circles stochastic simulations with delays for the DFM, with feedback delays sampled from. The orange symbols are the results forn=10, the brown symbols forn=100 and the red symbols forn=1,000. The black circles are simulations for the DFM with a fixed feedback delay, equivalent to the 'n=∞' limit. In (c), simulations of the DFM with fixed delay, corresponding ton=∞. Orange circles are simulations of the DFM with a feedback gainφ=0.2, brown circlesφ=0.4 and red circlesφ=0.6. The dashed lines are approximations of the value of the Fano factor at the plateau calculated from equation (14). In both (b) and (c), the errors are smaller than the symbols. Figure 2a displays numerical calculations of the stoichiometric delay coefficient from Lyapunov's matrix equation, equation (3), for a process including 100 synthesis steps. The first observation is that for most feedback gains and feedback delays the coefficient s d is much smaller than unity. Second, the figure confirms the behaviour anticipated from equation (9) in the lower part of the figure and from equation (10) in the upper left corner. Figure 2: Feedback-regulated molecular fluctuations. ( a ) The size of the stoichiometric delay coefficient s d for different feedback gains and feedback delays in the SFM with n =100. Macroscopic oscillations of the concentration appear with parameters in the white area. ( b , c ) Intrinsic noise measured by the Fano factor of the SFM and the DFM. In ( b ), the solid line is the LNA, the plus signs stochastic simulations of the SFM and the circles stochastic simulations with delays for the DFM, with feedback delays sampled from . The orange symbols are the results for n =10, the brown symbols for n =100 and the red symbols for n =1,000. The black circles are simulations for the DFM with a fixed feedback delay, equivalent to the ' n =∞' limit. In ( c ), simulations of the DFM with fixed delay, corresponding to n =∞. Orange circles are simulations of the DFM with a feedback gain φ =0.2, brown circles φ =0.4 and red circles φ =0.6. The dashed lines are approximations of the value of the Fano factor at the plateau calculated from equation (14). In both ( b ) and ( c ), the errors are smaller than the symbols. Full size image We exploit the Fano factor F = C rr /〈 X r 〉 to quantify the intrinsic noise. For the SFM, the Fano factor is numerically computed using equation (3). In addition, we measure the Fano factor from stochastic simulations of the SFM and the DFM, using a version of the stochastic simulation algorithm [14] for delayed reactions [12] , [13] . For the DFM simulations, the finite number of steps must be translated to an appropriate feedback delay, as the time τ i to take one step forward in the SFM is exponentially distributed and the expected time for a molecule to propagate from step 1 to step n is not exactly τ d , but rather follows a distribution with the mean and variance If the step rate is constant, κ I = κ , then it follows from (11) and (12) that the feedback delay is gamma distributed with mean τ d = n / κ and variance [19] . By the central limit theorem, the distribution of the total delay time is well approximated by the normal distribution when n grows. In the (artificial) limit n →∞ with a finite feedback delay, we obtain the delta distribution δ ( τ − τ d )—equivalent to an explicit-fixed feedback delay. When n =1, the delay is exponentially distributed. The distribution for the delayed events resulting from the SFM model can therefore be broad or very narrow depending on which n is used. The Fano factor computed from the LNA and the simulations are plotted in Figure 2b . First of all, it is clear that the feedback delay τ d must be smaller than unity for the feedback to suppress molecular fluctuations. In the original variables, this translates to feedback delays smaller than the average lifetime of the r-molecule t d <1/ b . A Fano factor greater than unity is a direct consequence of the stoichiometric delay coefficient, and the maximum is reached for feedback delays larger than the lifetime of the r-molecule. The decay for longer feedback delays can be explained by the increased width of the distribution of the feedback delay, which scales as . The positively correlated synthesis events generated by the feedback in the first biochemical step are smeared during the n steps and are therefore not apparent in the final stage of making the molecule. In the limit n →∞ and a fixed τ d >1, there is no increased width of the distribution of feedback delays, and therefore no decay in the stoichiometric delay coefficient. Therefore, the black circles from the DFM simulations in Figure 2b show a plateau rather than a peak. In this limit, the covariance or Fano factor can be calculated from the solution of an integral equation. The value at the plateau can be determined explicitly ( Supplementary Note 2 ). which implies that the stoichiometric delay coefficient in this limit is approximately s d ≈ φ 2 . In Figure 2c , we display the Fano factor from stochastic simulations of a fixed delayed feedback. The approximation in equation (13) is less accurate for larger feedback gains, but as we can see it holds well up to φ =0.6. The relation (13) can be understood intuitively by considering two independent, identically distributed, stochastic variables X and Y . For longer delays, the feedback control on X is then modelled by the (uncorrelated) influence of Y . It follows from ref. 20 that the relation between the Fano factors is ( Supplementary Note 2 ) As F X = F Y , we have that F X =1/(1− φ 2 /2) and (13) follows. Propagation of delay-induced fluctuations The consequences of delay-dependent intrinsic noise will of course depend on the biological context of the regulatory molecule. The systems responding to the fluctuating species will, however, in many cases have evolved to respond to the whole distribution of the fluctuating input and not just its average value. For this reason, the overall system dynamics will in some cases only seem rational when the fluctuations are considered in the analysis. 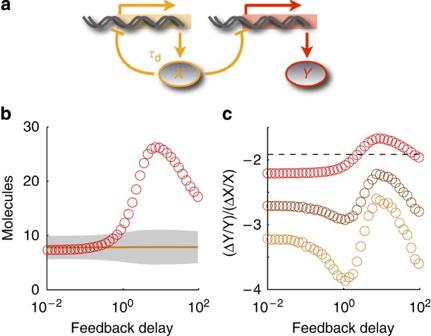Figure 3: Propagation of fluctuations. The panel (a) illustrates the auto-regulation ofXandX's regulation ofY. The auto-regulation is repressive and has the same properties as inFigure 2b, with feedback gainφ=0.75 andn=1,000 synthesis steps. The negative regulation ofYis modelled using a Hill functionF(X)=k/(1+(X/K)2). In (b), we plot the mean number ofXmolecules (orange line) and its deviation (shaded area). The red circle shows the mean number ofYmolecules, which is achieved usingK=〈X〉/50, the maximal ratek=α(equal maximum rate ofX). The decay rate constant ofYis 0.001. (c) Sensitivity amplification (ΔY/Y)/(ΔX/X)when perturbing the maximal rate ofXmolecules by 5%. From top to bottom,K=〈X〉/5, 〈X〉/25 and 〈X〉/50, with all other parameters as in (b). The dashed line is the large-molecule limit amplification, where 〈F(X)〉=F(〈X〉), calculated for a 5% perturbation, which is approaching −2 (the Hill coefficient) when the perturbation becomes infinitesimally small. To illustrate this point, we extend the autorepressor system to regulate the synthesis of another molecule, depicted in Figure 3a . The feedback regulation of the molecule X is the same as the one given in Figure 2b , with the same feedback gain. The regulation of the second molecule, Y , is repressive and modelled by F ( X )= k /(1+( X / K ) 2 ), where it is assumed that the X molecule equilibrates at its state of repression on a much faster timescale than the relaxation time of the distribution of X molecules, P ( X ). Under these conditions, the average synthesis rate of , which implies that the concentration of Y will depend on the fluctuations in X , as F ( X ) is a non-linear function and therefore 〈 F ( X )〉≠ F (〈 X 〉). To illustrate this point, we perform stochastic simulations of the biochemical reactions and the results are displayed in Figure 3b . The orange line is the mean level of X molecules, which does not depend on the feedback delay in the synthesis of X molecules, whereas the deviation from the mean value does, as is illustrated by the shaded area. The red circles are the mean number of Y molecules. The Y synthesis responds to the broadening of the X distribution, and the average number of Y therefore responds to the delay in X regulation, although the average number of X molecules does not. This effect can be tuned to any desired value by tuning the parameters. More interestingly, the sensitivity amplification for the regulation of Y by X , (Δ Y / Y )/(Δ X / X ) will increase for certain time delays as can be seen in Figure 3c . The sensitivity amplification is increased when a change in the average concentration generates a disproportionate response because of the non-linear response to the perturbed fluctuation profile—a phenomenon known as stochastic focusing [21] . Here with the result that Y is most sensitive to changes in X for time delays corresponding to the lifetime of X molecules, where the fluctuations are close to independent of the feedback and the noise is Poissonian. Figure 3: Propagation of fluctuations. The panel ( a ) illustrates the auto-regulation of X and X 's regulation of Y . The auto-regulation is repressive and has the same properties as in Figure 2b , with feedback gain φ =0.75 and n =1,000 synthesis steps. The negative regulation of Y is modelled using a Hill function F ( X )= k /(1+( X / K ) 2 ). In ( b ), we plot the mean number of X molecules (orange line) and its deviation (shaded area). The red circle shows the mean number of Y molecules, which is achieved using K =〈 X 〉/50, the maximal rate k=α (equal maximum rate of X ). The decay rate constant of Y is 0.001. ( c ) Sensitivity amplification (Δ Y / Y) /(Δ X/X) when perturbing the maximal rate of X molecules by 5%. From top to bottom, K =〈 X 〉/5, 〈 X 〉/25 and 〈 X 〉/50, with all other parameters as in ( b ). The dashed line is the large-molecule limit amplification, where 〈 F ( X )〉= F (〈 X 〉), calculated for a 5% perturbation, which is approaching −2 (the Hill coefficient) when the perturbation becomes infinitesimally small. Full size image Regulation is essential when it is desirable to maintain homoeostasis in a variable environment and because of intrinsic fluctuations at the molecular level also in a constant environment. Imprecise regulation is costly because it results in a deviation between the production and demand of the regulated species. Making too few molecules will limit downstream pathways or functions and making too many may lead to the fact that resources are wasted in maintaining too high intracellular pools, or worse, to toxic levels of the molecule. The feedback delay of indirect feedback is a result of the many consecutive steps when making a protein, mRNA, a metabolic product in many enzymatic steps or to process, modify and transport a macromolecule in the cell. As the feedback delay will have a significant influence on the dynamic and stochastic properties of the system, it has to be included in the design or evolution of the regulator system as well as in its analysis. For negative auto-repression to successfully repress fluctuations, the feedback delay has to be shorter than the timescale of relaxation of the regulated quantity. This may seem trivial to achieve for gene expression, as the typical relaxation timescale for stable proteins is in the order of the generation time of the cell. However, in many cases, the relaxation time of the regulated species can be much shorter than the generation time, such as in the case of RNA degradation [22] , metabolite turnover or proteolytic degradation of proteins. In these cases, fast feedback is essential or, as we just have seen, it may have deleterious effects. In this context, it is also important to remember that the feedback delay will change with the environmental conditions. For instance, under amino-acid starvation, the time required to synthesize a protein may be significantly delayed because of ribosomal stalling. A robust feedback system must therefore handle variations in the mean feedback delay and its distribution. For example, the feedback should not induce oscillations when the feedback delays are unusually lengthy, which requires a moderate feedback gain. Even if the feedback gain does not promote oscillations, anomalously large fluctuations may occur for intermediate time delays. 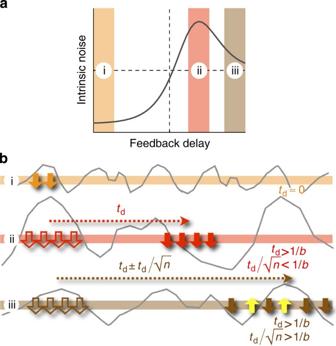Figure 4: Summary of the feedback response for various feedback delays. (a) The intrinsic noise and (b) illustrations of the different feedback responses. The dashed horizontal line inais the noise level of unregulated synthesis, and the dashed vertical line is positioned at the lifetime of the r-molecule. When the feedback delay is short (i), the regulation is direct and anticorrelated with the deviation from the stationary concentration. The result is less noise and a shorter timescale of variations because of a faster relaxation to the stationary concentration. In this example, the relaxation time is approximately half of the lifetime of the r-molecule and the variance is approximately half of the average number of molecules. For intermediate feedback delays (ii), the relaxation time is approximately equal to the lifetime of the r-molecule, which sets the correlation time of the feedback regulation (open arrows). The delayed responses (solid arrows) are released at time points with concentrations not correlated with the direction of the responses. The result is synthesis bursts, which generate larger fluctuations from the stationary concentration—in this example, a variance∼50% larger than the average number of molecules. For long feedback delays (iii), the feedback regulation is correlated on the same timescale as in ii. The deviation in the synthesis time is, however, broadened and synthesis events are mixed with each other, which diminish the correlations in the feedback regulation. In this situation, the noise is equivalent to that of an unregulated synthesis of molecules, where the variance is approximately equal to the average number of molecules. Figure 4 summarizes the feedback response for various feedback delays. For short feedback delays, shorter than the lifetime of the r-molecule, the feedback will counteract the deviations from the steady state and thus reduce fluctuations, as illustrated by (i). This noise-reducing effect will be reached independently of the number of consecutive synthesis steps. When the feedback delay is longer than the lifetime of the regulated species, the delayed response will change the state in a random direction as compared with the current deviation from the steady state and the noise-reducing effect of feedback is lost, (ii) and (iii). Moreover, although the synthesis of new molecules is uncorrelated to the current state, the signal to the feedback is correlated on the timescale of fluctuations of the r-molecule, which for large feedback delays is 1/ b —the lifetime of the r-molecule. Therefore, the feedback generates periods of increased activity, where the synthesis events lie close in time and effectively resulting in stoichiometries larger than one. For fixed feedback delays, the feedback-regulated synthesis events and their associated stoichiometries are transferred in time, unchanged, to the synthesis of molecules and thus remains no matter how long the feedback delay is. If, on the other hand, the feedback delay is a result of a finite number of consecutive synthesis steps, any feedback-generated correlations on the first synthesis step will be translated to the synthesis of r-molecules for intermediate feedback delays (ii) but vanish for longer synthesis times (iii). The reason is the deviation in the synthesis time, which scales as . For long feedback delays, , new molecules will, as a result of the increased deviation in the synthesis time, be created independently—equivalent to production without feedback, thus displaying Poissonian statistics. We conclude that distributed feedback delays that arise from a limited number of consecutive enzymatic steps in general result in a more robust feedback regulation than a sharp fixed feedback delay, as the distributed delay makes the system forget obsolete regulatory actions. We note that the reason many feedback processes occasionally will run into long feedback delays is the limitation of one of several key metabolites, such as 1 amino acid out of 20, a coenzyme in anabolic reactions. In these cases, the distribution of the feedback delay will be broad, because it is only one or a few steps in the delay processes that are extended, and the negative effects of delayed feedback regulation will be mild. We also note that there are processes that will accentuate the positive correlation between delayed events, such as queuing of stalled RNA polymerase and ribosomes. Such effects will result in even larger effective stoichiometries and more fluctuations. An accurate description of the dynamic distribution of delayed events in these cases will require numerical simulations that go beyond the analytical results presented in this study. Finally, although the anomalously large fluctuations observed at intermediate time delays by definition are counterproductive in terms of maintaining homoeostasis, the fluctuation may still have positive contributions when seen in a broader perspective. For example, we have shown that the auto-repressed species may be a more potent regulator of a downstream process when the delay-induced fluctuations are taken into account. In closing, both distributions of fluctuations and time delays are evolved together with all other properties of the systems. It is therefore expected that several aspects of intracellular regulation only make sense when time delays and stochastic processes are included in the analysis. Figure 4: Summary of the feedback response for various feedback delays. ( a ) The intrinsic noise and ( b ) illustrations of the different feedback responses. The dashed horizontal line in a is the noise level of unregulated synthesis, and the dashed vertical line is positioned at the lifetime of the r-molecule. When the feedback delay is short (i), the regulation is direct and anticorrelated with the deviation from the stationary concentration. The result is less noise and a shorter timescale of variations because of a faster relaxation to the stationary concentration. In this example, the relaxation time is approximately half of the lifetime of the r-molecule and the variance is approximately half of the average number of molecules. For intermediate feedback delays (ii), the relaxation time is approximately equal to the lifetime of the r-molecule, which sets the correlation time of the feedback regulation (open arrows). The delayed responses (solid arrows) are released at time points with concentrations not correlated with the direction of the responses. The result is synthesis bursts, which generate larger fluctuations from the stationary concentration—in this example, a variance ∼ 50% larger than the average number of molecules. For long feedback delays (iii), the feedback regulation is correlated on the same timescale as in ii. The deviation in the synthesis time is, however, broadened and synthesis events are mixed with each other, which diminish the correlations in the feedback regulation. In this situation, the noise is equivalent to that of an unregulated synthesis of molecules, where the variance is approximately equal to the average number of molecules. Full size image Calculating the covariance matrix Given a Jacobian matrix A and a diffusion matrix V , the steady-state covariance matrix C is in the LNA of a biochemical reaction network at a fixed point (without feedback delay) obtained from Lyapunov's matrix equation (3). The LNA describes the covariance exactly if the feedback Φ is linear in x r . Otherwise, it is an approximation. The Jacobian matrix is calculated from the differential equation (1) describing the rate of change of the mean values of the different species in the multistep synthesis and is evaluated at the stationary point x s ( Supplementary Note 1 ). For simplicity, we have assumed equal step rates κ i = κ . The diffusion matrix is given by the frequency of reactions and their corresponding stoichiometries at the stationary point x s , where a l is the rate of reaction l , v li the stoichiometric coefficient for element i in reaction l and δ ij is the Kronecker delta [23] . The mean number of r-molecules is 〈 X r 〉= x r , s . We obtain, using that αΦ [ x r, s ]= x r, s at the stationary solution when i = j =1, Now, assume that equation (3) has a solution of the form The variable γ is yet to be determined. Inserting the above ansatz into equation (3) will verify the consistency of the ansatz and that all elements satisfy , where m is a constant, independent of κ and φ , with a magnitude of the order of unity. The advantage of rewriting C in terms of γ as described above is that the ansatz captures the major influence of φ and κ on the solution, and will therefore render expressions that nicely display the effects of different feedback gains and feedback delays. For more details, see Supplementary Note 2 . How to cite this article: Grönlund, A. et al . Delay-induced anomalous fluctuations in intracellular regulation. Nat. Commun. 2:419 doi: 10.1038/ncomms1422 (2011).